Complete quantum control of exciton qubits bound to isoelectronic centres In recent years, impressive demonstrations related to quantum information processing have been realized. The scalability of quantum interactions between arbitrary qubits within an array remains however a significant hurdle to the practical realization of a quantum computer. Among the proposed ideas to achieve fully scalable quantum processing, the use of photons is appealing because they can mediate long-range quantum interactions and could serve as buses to build quantum networks. Quantum dots or nitrogen-vacancy centres in diamond can be coupled to light, but the former system lacks optical homogeneity while the latter suffers from a low dipole moment, rendering their large-scale interconnection challenging. Here, through the complete quantum control of exciton qubits, we demonstrate that nitrogen isoelectronic centres in GaAs combine both the uniformity and predictability of atomic defects and the dipole moment of semiconductor quantum dots. This establishes isoelectronic centres as a promising platform for quantum information processing. Isoelectronic centres (ICs) are atomic-sized defects that were first identified and studied several decades ago [1] . They are formed from one, two or a small number of isovalent impurities in a semiconductor. The IC investigated in this work is composed of two nitrogen atoms positioned substitutionally on the GaAs anionic sublattice as presented in Fig. 1a . 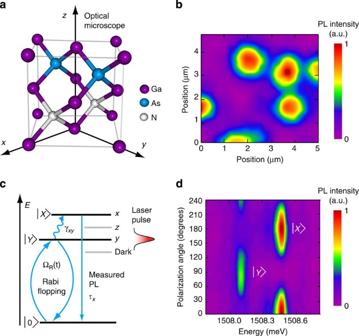Figure 1: Nitrogen pairs and coherent control scheme. (a) Nitrogen pairs ofC2vsymmetry in first anionic nearest-neighbour configuration. (b) 5 μm × 5 μm off-resonance PL intensity map of nitrogen pairs in GaAs at 1.508 eV, showing that single nitrogen pairs are spatially resolved. (c) Schematic representation of the excitonic fine structure of nitrogen pairs ofC2vsymmetry along with the emission polarization from each state. To achieve coherent control of the exciton, Rabi oscillations between the ground state |0› and the exciton state |Y› are driven at a frequency ΩR(t). The population of |Y› is obtained by measuring the luminescence from the cross-polarized state |X›. The transfer rate between the two states isγyxand the characteristic time decay of the PL isτx. (d) Off-resonance polarization-resolved PL spectra of excitons bound to a single nitrogen pair, showing two linearly polarized transitions. Figure 1: Nitrogen pairs and coherent control scheme. ( a ) Nitrogen pairs of C 2v symmetry in first anionic nearest-neighbour configuration. ( b ) 5 μm × 5 μm off-resonance PL intensity map of nitrogen pairs in GaAs at 1.508 eV, showing that single nitrogen pairs are spatially resolved. ( c ) Schematic representation of the excitonic fine structure of nitrogen pairs of C 2v symmetry along with the emission polarization from each state. To achieve coherent control of the exciton, Rabi oscillations between the ground state |0› and the exciton state | Y › are driven at a frequency Ω R ( t ). The population of | Y › is obtained by measuring the luminescence from the cross-polarized state | X ›. The transfer rate between the two states is γ yx and the characteristic time decay of the PL is τ x . ( d ) Off-resonance polarization-resolved PL spectra of excitons bound to a single nitrogen pair, showing two linearly polarized transitions. Full size image The physics of ICs is reminiscent of quantum dots (QDs), a system widely studied for quantum computation [2] , [3] , [4] , [5] , [6] . Their semiconductor host allows one to take advantage of convenient optical selection rules for spin initialization, manipulation and readout; to exploit dynamic charge doping, electrical coherent control [7] and device integration; and to fabricate high quality Bragg reflectors and cavities. Just like QDs, ICs can trap multiple charge configurations: single electrons (or holes for pseudo-donors like Te in ZnSe), excitons, biexcitons and charged excitons [8] . The latter could be used to take advantage of the powerful single spin quantum control schemes demonstrated in QDs [2] . Finally, there exist many isoelectronic centre/host systems and a number of these centres have been spatially resolved and individually studied: N in GaAs [9] and GaP [10] ; and Te in ZnSe [11] . The atomic nature of ICs is also reminiscent of phosphorus dopants in silicon, in which single qubit gates were realized [12] , and NV centres in diamond, in which two-qubit gates and distant spin entanglement have been demonstrated [13] , [14] . Shrinking semiconductor nanostructures to the size of a few impurities provides the predictability and uniformity of these atomic defects. Owing to a confinement potential and symmetry perfectly defined by the few substitutional sites involved within the host crystal lattice, any configurational variation leads to a radical modification of electronic states and large discrete variation of the emission energy. Therefore, by spectrally selecting a single configuration, configurational broadening, which is very important for QDs, is suppressed. Inhomogeneous broadening is then limited to the environmental disorder set by the host material quality and purity. For the nitrogen pair configuration shown in Fig. 1a , large-ensemble photoluminescence (PL) measurements reveal an inhomogeneous broadening lower than 25 GHz [15] , which is comparable to that of NV centres and other atomic defects [16] , [17] . This high optical homogeneity is of strategic importance as it reduces the implementation complexity of quantum processing schemes. In this work, resonant PL of excitons bound to N pairs in GaAs is measured. Through Rabi rotations of the exciton, we show that the high homogeneity of ICs is complemented by an optical dipole moment comparable to that of QDs [18] and higher than that of NV centres [19] . This should allow strong coupling with a cavity, which is a key property for the realization of large-scale optical interconnection of distant qubits and robust quantum networks [20] , [21] . Moreover, the complete quantum control of exciton qubits is demonstrated by Ramsey interferometry, establishing ICs as a promising platform for quantum information processing. Resonant PL The coherent control of excitons is realized on single nitrogen pairs using confocal microscopy. The PL intensity map of Fig. 1b shows spatially resolved nitrogen pairs emitting at 1.508 eV. The excitonic fine structure reveals emitters of C 2v symmetry and empirical pseudopotential calculations indicate a first anionic neighbour configuration [22] . For the measurement configuration shown in Fig. 1a , two transitions are forbidden (dark) and two others are inaccessible ( z ), such that only four linearly polarized transitions are expected in a strain free host [23] (see Supplementary Note 1 and Supplementary Table 1 ). However, the sample used in this study was grown at suboptimal temperatures to intentionally generate crystal imperfections and strain fields affecting the relative strength of the crystal field and exchange interactions defining the excitonic fine structure. In this case, similar to the case of strained QDs where light- and heavy-hole degeneracy is lifted, four excitonic transitions are pushed to higher energy and only four remain, as shown schematically in Fig. 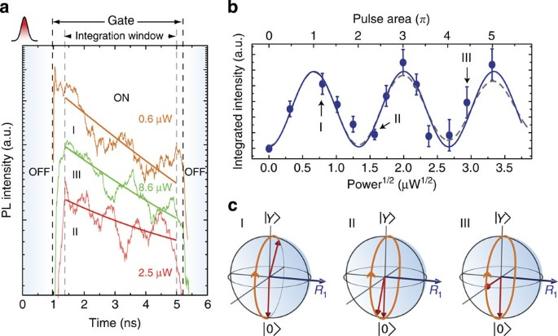Figure 2: Rabi rotations. (a) Time-correlated resonant PL intensity from |X› for 3 excitation powers, showing an exponential decay fitted with the characteristic timeτx=3.9 ns. The detector is gated 1 ns after the laser pulse to discriminate the PL signal from the strong control pulse. (b) Resonant PL integrated intensity as a function of the square root of the control laser power. The points identified by labels I, II and III correspond to the data presented ina. The solid line was fitted without considering any damping caused by EID. The dashed curve represents a fit of the data with an EID damping coefficient ofK2=4 fs. Error bars are established from the range of intensities satisfactorily fitting PL decay curves. (c) Bloch vector trajectories in the rotating frame for the three powers shown ina. The red arrows represent the initial and final states andR1is the axis of rotation. 1c (see Supplementary Table 2 ). Of these four transitions, only two bright linearly polarized states | X › and | Y › can be measured, as seen from the polarization-resolved PL spectrum presented in Fig. 1d . Resonant PL is measured using the experimental scheme presented in Fig. 1c . A linearly polarized control pulse is tuned in resonance to drive Rabi oscillations between the ground state |0› (no exciton) and the state | Y › at a frequency Ω R ( t )= μE ( t )/ ℏ , where μ is the exciton dipole moment and E ( t ) the amplitude of the electric field. The population created in | Y › is partially transferred at a rate γ yx to the cross-polarized state | X › from which the PL intensity is measured using a fast-gated single-photon avalanche diode (SPAD) [24] . Hyperfine interaction is believed to be the dominant transfer mechanism between | Y › and | X › as spin relaxation due to spin–orbit interaction or the Bir–Pikus hamiltonian are quenched for strongly confined excitons [25] , [26] . This mechanism does not couple | Y › and | X › directly and γ yx will thus depend on all possible transfer rates between bright excitons, | X › and | Y ›, and dark excitons, | Z › and | D › (see Supplementary Note 2 ). Figure 2a shows the time-correlated resonant PL at different excitation powers. Every curve is fitted with a monoexponential decay with the same characteristic time τ x =3.9 ns and with a varying background signal originating from residual laser noise. The characteristic time is the result of a complex dynamic governed by all possible transfers between the four exciton states and their radiative emission (see Supplementary Note 2 and Supplementary Fig. 1 ). The total PL intensities are obtained by integrating the fitted curves over the window defined in Fig. 2a . Figure 2: Rabi rotations. ( a ) Time-correlated resonant PL intensity from | X › for 3 excitation powers, showing an exponential decay fitted with the characteristic time τ x =3.9 ns. The detector is gated 1 ns after the laser pulse to discriminate the PL signal from the strong control pulse. ( b ) Resonant PL integrated intensity as a function of the square root of the control laser power. The points identified by labels I, II and III correspond to the data presented in a . The solid line was fitted without considering any damping caused by EID. The dashed curve represents a fit of the data with an EID damping coefficient of K 2 =4 fs. Error bars are established from the range of intensities satisfactorily fitting PL decay curves. ( c ) Bloch vector trajectories in the rotating frame for the three powers shown in a . The red arrows represent the initial and final states and R 1 is the axis of rotation. Full size image Rabi rotations Rabi rotations are first demonstrated using this resonant PL scheme. Figure 2b displays the integrated PL intensity measured as a function of the square root of the control laser power, which is proportional to the pulse area θ =∫Ω R ( t ) dt . This control pulse rotates the qubit by an angle θ about the axis R 1 on the Bloch sphere, as shown in Fig. 2c . Hence, for a π (2 π ) pulse, the system is brought to the eigenstate | Y › (|0›) and the PL from | X ›, directly proportional to the population of | Y ›, will be maximal (minimal). The sinusoidal dependence of the measured PL intensity is a clear signature of Rabi oscillations. From the period of Rabi rotations fitted in Fig. 2b , an exciton dipole moment of 65±28 D is extracted. Measurements from several nitrogen pairs revealed dipole moments ranging from 5 to 65 D (see Supplementary Fig. 2 ) with an overall average of 27 D. We believe that the large variation in dipole moment is not intrinsic to ICs, but is due to the local strain fields deliberately introduced in our sample. These are comparable to dipole moments obtained from InGaAs QDs and thickness fluctuation QDs in GaAs quantum wells. For InGaAs QDs, single particle confinement energies dominate excitonic effects and measured dipole moments range from 10 to 40 D [27] , which are consistent with models assuming weak electron-hole correlation [28] . The lateral size of thickness fluctuation QDs generally exceeds the exciton Bohr radius such that both excitonic effects and the large exciton wavefunction can enhance the oscillator strength [29] . Dipole moments up to 75 D have been reported in this system [18] , about twice those of InGaAs QDs. According to the prevalent model of excitonic binding to ICs [1] , [22] , the electron is confined to the nitrogen core potential while the hole is bound to the electron by Coulomb interaction, which is weakened by repulsion from the nitrogen core. This binding mechanism implies that excitonic effects could play a significant role in explaining the large dipole moment observed. Interestingly, the amplitude of Rabi oscillations is preserved over nearly three complete rotations, indicating that ICs are not subject to the important excitation-induced dephasing (EID) consistently encountered in QDs. EID increases with excitation power and can be modelled by a dephasing rate Γ 2 = K 2 Ω R ( t ) 2 , where coefficient K 2 should be minimal to preserve the fidelity of qubit manipulations. The results of Fig. 2b are best fitted without any EID ( K 2 ~0), but taking into account the estimated errors on the PL intensity, an upper bound of K 2 ≤4 fs is estimated (see dashed curve). The coupling of excitons to longitudinal-acoustic phonons, which is proportional to the square of the exciton deformation potential, has been proposed as a dominant EID mechanism [30] . In ICs, the tight localization of the electron wavefunction reduces the deformation potential to 3.7 eV (ref. 31 ) in comparison with 9 eV for QDs. Therefore, EID caused by longitudnal-acoustic phonons is expected to be six times less important in our system, in very good agreement with our experimental results. Ramsey interference To show that excitons bound to ICs are useable qubits, we demonstrate their complete quantum control over the Bloch sphere and measure their coherence time by Ramsey interferometry. Two π /2 pulses are tuned in resonance with the exciton transition and delayed by τ = τ c + τ f , where τ c and τ f represent respectively coarse and fine time delays ( Fig. 3a ). As shown in Fig. 3b , the first pulse brings the quantum state on the equatorial plane of the Bloch sphere and the second pulse causes a rotation of π /2 about the axis defined by (cos?, sin?, 0), where ?= ωτ is the phase acquired by the exciton. By selecting the delay, a rotation on the Bloch sphere about an arbitrary axis can be realized. 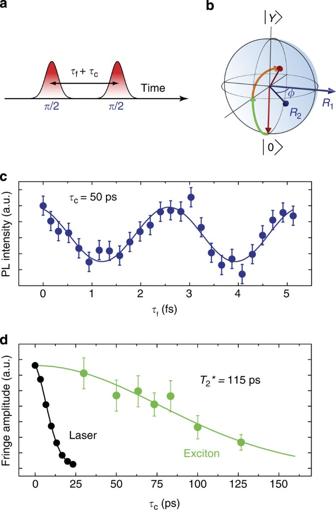Figure 3: Ramsey interference. (a) Pulse sequence for Ramsey interference: twoπ/2 pulses with a delay ofτ=τf+τcexcite the exciton. (b) Bloch vector trajectory in the Ramsey interference experiment in the rotating frame. The first pulse rotates the Bloch vector about the axisR1. The second rotation is about the axisR2defined by the angle ?=ωτ. Red arrows represent the initial and final excitonic states. (c) PL intensity as a function of the fine delayτfforτc=50 ps. Intensities are obtained by fitting time-resolved PL curves with a monoexponential decay. Error bars indicate the range of acceptable intensity values. The solid line represents a sinusoidal fit of the data. (d) Amplitude of Ramsey fringes as a function of the coarse delayτcalong with the autocorrelation function of the laser. Error bars indicate the range of acceptable amplitudes obtained from sinusoidal fits similar to the one presented inc. Solid lines are Gaussian fits of the data. An exciton coherence time ofps is extracted. Figure 3: Ramsey interference. ( a ) Pulse sequence for Ramsey interference: two π /2 pulses with a delay of τ = τ f + τ c excite the exciton. ( b ) Bloch vector trajectory in the Ramsey interference experiment in the rotating frame. The first pulse rotates the Bloch vector about the axis R 1 . The second rotation is about the axis R 2 defined by the angle ?= ωτ . Red arrows represent the initial and final excitonic states. ( c ) PL intensity as a function of the fine delay τ f for τ c =50 ps. Intensities are obtained by fitting time-resolved PL curves with a monoexponential decay. Error bars indicate the range of acceptable intensity values. The solid line represents a sinusoidal fit of the data. ( d ) Amplitude of Ramsey fringes as a function of the coarse delay τ c along with the autocorrelation function of the laser. Error bars indicate the range of acceptable amplitudes obtained from sinusoidal fits similar to the one presented in c . Solid lines are Gaussian fits of the data. An exciton coherence time of ps is extracted. Full size image Figure 3c shows Ramsey fringes in the relative PL intensity from the state | X › as the fine time delay τ f between the two pulses is swept while the coarse delay is kept constant at 50 ps. To unambiguously demonstrate that quantum interference is realized, the amplitude of Ramsey fringes is shown in Fig. 3d as a function of the coarse delay along with the autocorrelation function of the laser pulse. The interference amplitude of the laser decays with a time constant of 15 ps, an order of magnitude shorter than the time decay of the Ramsey fringes, which is best fitted by a gaussian function with a coherence time of ps. This coherence time is similar or slightly higher than coherence times of excitons bound to QDs [27] , [32] . The gaussian decay is a signature of non-markovian dephasing, characterized by a reservoir relaxation rate slower than the decoherence rate of the two-level quantum system. Environmental fluctuations in the vicinity of the nitrogen pair can affect the evolution of the exciton wavefunction and could explain the non-markovian decoherence observed [4] . Complete coherent control of excitons bound to nitrogen ICs in GaAs was demonstrated through Rabi rotations and Ramsey interferometry. The combination of high optical homogeneity and a large dipole moment could prove to be crucial ingredients for large-scale photonic integration of two-qubit gates, making ICs a promising alternate platform for quantum computation. For exciton qubits, low EID allows faster qubit manipulation that could lead to the threshold for fault-tolerant quantum computation within the relatively short lifetime. Although the operating temperature of the exciton qubit demonstrated here is limited to 15 K, higher temperatures are expected from nitrogen ICs located deeper in the gap of GaAs [22] . Furthermore, the large exciton-binding energies found in wider gap materials (for example, N pairs in GaP [1] , [33] and Te pairs in ZnSe [11] ) should provide operating temperatures similar to those of epitaxial QDs. It appears relevant to investigate the impurity-host systems providing the optimal characteristics for quantum information processing. Finally, ICs are also well adapted for longer lived qubits like electron spins, as the existence of negatively charged excitons allows exploiting the control schemes already developed for QDs. Sample growth The sample was grown by molecular beam epitaxy and is composed of a 25 nm GaAs:N layer clad by 5 nm layers of GaAs and sandwiched between two Al 0.25 Ga 0.75 As barriers. Resonant PL measurements Microluminescence measurements are carried out in a custom made confocal microscope inserted into a closed-looped cryostat at 4 K. Nitrogen pairs are located using a 780 nm CW laser coupled to an optical fibre. Excitons are then optically driven at a rate of 40 MHz using a Ti:sapphire laser tuned in resonance with one of the exciton states and coupled to the same optical fibre. Pulses of ~1 ps and ~15 ps are used to drive Rabi oscillations and similar results are obtained for both pulse widths. The 15 ps pulses are generated by spectrally filtering 100 fs pulses using a diffraction grating in a 2 f configuration with the optical fibre. The weak PL signal and the strong control laser are discriminated in time using a fast-gated SPAD [24] , [34] . The detector is kept off when hit by the control laser and then rapidly turned on (in less than 200 ps) to maximize the detected PL signal. Nine orders of magnitude of control light are suppressed by gating the SPAD 1 ns after the excitation pulse and by cross-polarized PL detection. For Rabi rotations measurement, a linear increase of PL intensity with excitation power originating from afterpulsing effect due to carriers trapped in the SPAD detector was substracted from the data. This afterpulsing effect is also responsible for larger error bars in Fig. 2c at higher laser power. Ramsey interference Ramsey interferometry was realized by generating pairs of 15 ps pulses of controllable delay with a phase-stabilized Michelson interferometer. The coarse delay is controlled by a motorized delay stage and the fine delay by a piezoelectric positioner. The stabilization of the interferometer provides a resolution better than 0.1 fs on the fine delay. The presented PL intensities are relative to the intensity at τ f =0 fs. How to cite this article: Éthier-Majcher, G. et al. Complete quantum control of exciton qubits bound to isoelectronic centres. Nat. Commun. 5:3980 doi: 10.1038/ncomms4980 (2014).